Stochastic formation of magnetic vortex structures in asymmetric disks triggered by chaotic dynamics The non-trivial spin configuration in a magnetic vortex is a prototype for fundamental studies of nanoscale spin behaviour with potential applications in magnetic information technologies. Arrays of magnetic vortices interfacing with perpendicular thin films have recently been proposed as enabler for skyrmionic structures at room temperature, which has opened exciting perspectives on practical applications of skyrmions. An important milestone for achieving not only such skyrmion materials but also general applications of magnetic vortices is a reliable control of vortex structures. However, controlling magnetic processes is hampered by stochastic behaviour, which is associated with thermal fluctuations in general. Here we show that the dynamics in the initial stages of vortex formation on an ultrafast timescale plays a dominating role for the stochastic behaviour observed at steady state. Our results show that the intrinsic stochastic nature of vortex creation can be controlled by adjusting the interdisk distance in asymmetric disk arrays. Controlling fluctuations such as Barkhausen noise in ferro- and antiferro-magnetic materials require a fundamental understanding of non-deterministic phenomena [1] , [2] , [3] , [4] , [5] , [6] , [7] , [8] . As the length scales in nanomagnetism approach fundamental limits such as the exchange lengths, the question arises, whether there is an intrinsic stochastic nature, which ultimately would tremendously affect the performance of high-density magnetic storage devices aiming at faster processing speed. Understanding and controlling stochastic behaviour in nanoscale magnetic systems are thus a topic of paramount interest and numerous studies have been performed, for example, on magnetization reversal of nano-size domains in ultrathin magnetic films [5] , [8] , [9] and domain wall motion in magnetic nanowires [7] , [10] , [11] . The magnetic vortex is characterized by an in-plane circulating domain structure, the circularity c , which rotates either clockwise (CW, c =+1) or counter-clockwise (CCW, c =−1) and an out-of-plane magnetization, the polarity p pointing either up ( p =+1) or down ( p =−1) [12] , [13] , [14] , [15] , [16] , [17] , [18] . In the context of skyrmions, the magnetic vortex structure (VS) can be described by a topological charge, the skyrmion number of np /2=±1/2 with the winding number of n = ∮ [ α ( φ )/2π] d S=+1 (refs 19 , 20 , 21 ). Recently, magnetic VSs combined with perpendicular materials have been proposed to generate skyrmionic materials at room temperature [22] . This approach would open a route for practical uses of skyrmions [23] , [24] , [25] , [26] , [27] , [28] , [29] , which have so far been hampered by requirements such as specific crystal symmetries and low temperature [24] , [28] . A comprehensive investigation of stochasticity in the vortex formation and the clarification of its origin are essential particularly within closely packed arrays of nanodisks for achieving such skymionic structures and also for novel applications of VSs, but they have not been addressed so far. Here we report a systematic experimental and simulation study on the stochastic nature in the formation process of VSs in asymmetrically shaped permalloy (Ni 80 Fe 20 , Py) disks. A-priori , one would assume that only one type of circularity in asymmetrically shaped disks would be reliably selected as long as the direction of external fields for saturating and releasing the disks is fixed [30] , [31] , [32] , [33] . However, our results show that the final outcome of circularity depends on minute details of the dynamics in the initial stage of the formation process. We have used full-field magnetic transmission soft X-ray microscopy (MTXM) at the Advanced Light Source in Berkeley, CA, providing a spatial resolution of better than 25 nm to image the magnetic structures in asymmetric Py disks in their steady state [34] . The experimental details are described in the Methods section. Micromagnetic simulations, which take into account the onset time of the formation process, are used to interpret the observed steady-state configurations. 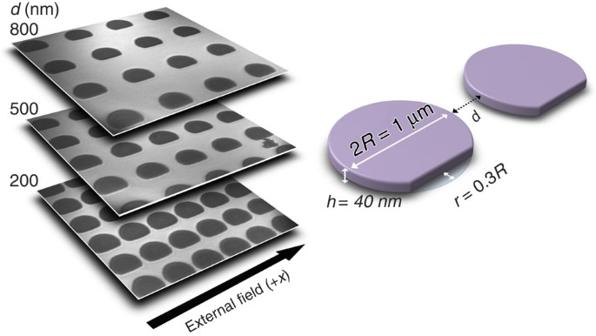Figure 1: Arrays of asymmetric Py disks with different interdisk distances. Schematic diagram of two neighbouring disks together with raw MTXM images for the arrays consisting of asymmetric disks with a radius ofR=500 nm, a height ofh=40 nm, an asymmetry ratio ofr=0.3Rand interdisk distances ofd=200, 500 and 800 nm are shown. Direct observation of magnetic VSs Figure 1 shows schematically the geometrical parameters for the asymmetric disks as well as raw MTXM images for the set of arrays studied. With a radius of R =500 nm, a height h =40 nm and an asymmetry ratio r =0.3 R , the interdisk distance was varied between d =200, 500 and 800 nm. An external magnetic field was applied parallel to the flat edges of the disks in + x direction to magnetically saturate the disks. To generate a VS, the disks were fully saturated at a field of +1 kOe and then immediately released to zero field without applying any external field in between saturation and remanent states. In Fig. 2a , representative images of in-plane domain structures taken from two successive measurements in the arrays of d =200, 500 and 800 nm are displayed. Repeated images were recorded at the same area of each array under identical measurement conditions. To enhance magnetic contrast and eliminate non-magnetic background, each image was normalized to a reference image taken at saturation state. As a result of the normalization procedure, the spin textures with in-plane domain structures rotating CW or CCW corresponding to c =+1 or c =−1 are clearly identified in Fig. 2a . As can be seen in the images, the generated circularity c in individual disks is not always the same within repetitions, but exhibits a stochastic character, particularly in the disks of d =500 nm, which is in sharp contrast to the assumption in previously published literatures that a certain circularity would be reliably formed in such disks because of the asymmetric geometry [30] , [31] , [32] . Interestingly, although the vortices were formed under an identical sequence of field sweep from +1 kOe to 0, CCW circularities ( c =−1) are predominantly generated in the disks within the array of d =200 nm, whereas CW circularities ( c =+1) are dominantly created in the disks with d =800 nm. On the other hand, there is no clear preference for any given circularity in the array with d =500 nm. The transition of predominantly created circularity from c =−1 to c =+1 by changing the interdisk distance from d =200 nm to d =800 nm is completely unexpected as a CW circularity has been reported to be formed in the same field sequence from +1 to 0 kOe in previous studies for the circularity control in asymmetric disks [30] , [31] , [32] . Micromagnetic simulations for the energies of CW and CCW vortex configurations show that the energy difference between CW and CCW states is very small (~10 −32 J) and comparable to the level of computational errors in all arrays regardless of the interdisk distance. Therefore, the observed phenomena cannot be explained by the energy difference between CW and CCW vortex states because of the asymmetric shape of disk. Figure 1: Arrays of asymmetric Py disks with different interdisk distances. Schematic diagram of two neighbouring disks together with raw MTXM images for the arrays consisting of asymmetric disks with a radius of R =500 nm, a height of h =40 nm, an asymmetry ratio of r =0.3 R and interdisk distances of d =200, 500 and 800 nm are shown. 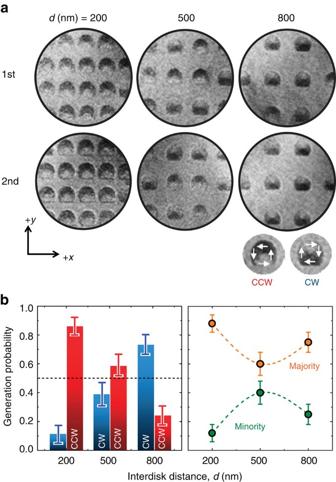Figure 2: Experimental observation of vortex structures in asymmetric Py disk arrays. (a) MTXM images of in-plane magnetic components taken from two successive measurements with the field sweep from +1 kOe to 0 in the arrays with various interdisk distances. The direction of magnetization is indicated by arrows in the two attached disk images. (b) The generation probabilities of CW and CCW circularities (majority and minority) as a function of the interdisk distance in left (right) panel. The values are obtained by statistical analysis of generation probabilities taken from 1,000 events (40 repeated measurements, 25 disks) for each array. The error bars indicate the full value of the standard deviation (s.d.) of generation probabilities from the statistical ensemble of 1,000. Full size image Figure 2: Experimental observation of vortex structures in asymmetric Py disk arrays. ( a ) MTXM images of in-plane magnetic components taken from two successive measurements with the field sweep from +1 kOe to 0 in the arrays with various interdisk distances. The direction of magnetization is indicated by arrows in the two attached disk images. ( b ) The generation probabilities of CW and CCW circularities (majority and minority) as a function of the interdisk distance in left (right) panel. The values are obtained by statistical analysis of generation probabilities taken from 1,000 events (40 repeated measurements, 25 disks) for each array. The error bars indicate the full value of the standard deviation (s.d.) of generation probabilities from the statistical ensemble of 1,000. Full size image Stochasticity in the formation of VSs To systematically investigate the stochastic behaviour in the formation of circularity and the change of dominantly created circularity as a function of the interdisk distance, we accumulated statistical data from repeated measurements of the vortex formation more than 40 times and checked the VSs in 25 individual disks, which gives a statistical ensemble of 1,000 events in each array. Figure 2b summarizes the generation probabilities of CW and CCW circularities in the arrays with different interdisk distances where the error bars indicate the standard deviations in the generation probabilities of 25 disks. To clearly visualize the stochasticity in the circularity formation, we plot in the right column of Fig. 2b the generation probabilities of majority and minority states, which are dominantly and recessively created circularities in the repeated measurements. The degree of stochasticity is complementary to the concept of repeatability for the creation of the identical circularity. Thus, a higher generation probability of majority states corresponds to a lesser degree of stochasticity in the formation process. Most notably, there seems to be a strong correlation between stochasticity and interdisk distance. The disk array with d =500 nm shows higher stochasticity and no significant differences between majority and minority probabilities than the arrays with the shorter ( d =200 nm) and the longer interdisk distance ( d =800), which is shown as V-shaped graphic chart in the generation probability of majority (see right column in Fig. 2b ). From those measurements, the transition of dominantly created circularity from c =−1 to c =+1 with increasing the interdisk distance is also evident. The experimentally observed phenomena, particularly the V-shaped dependency of stochasticity on the interdisk distance is very intriguing as it cannot originate from thermal fluctuation effect, which has been considered as the main cause of stochastic behaviour in magnetic processes [9] , [10] , [11] . Thermal fluctuations should not depend on the interdisk distance because the thermal fluctuations (~ k B TV −1 ) (refs 35 , 36 ) are mainly determined by the temperature T and the island volume V , the unit volume relevant to thermal stability and not by geometrical parameters, such as the interdisk distance. Micromagnetic simulations for the vortex creation To understand the origin of the dependence of stochasticity with the interdisk distance, we performed micromagnetic simulations for the vortex formation in asymmetrically shaped disks. In this simulation, we deliberately excluded thermal noise to extract non-thermal contributions, which trigger the observed phenomenon in Fig. 2 . We used the OOMMF code (see http://math.nist.gov/oommf ), which is based on the Landau–Lifshitz–Gilbert equation [37] , [38] for the local magnetization vector M ( r ): δ M / δt =− γ ( M × H eff )+ α /| M |( M × δ M/ δt ) with the phenomenological damping constant α, the gyromagnetic ratio γ and the effective field H eff . Standard material parameters for Py were used for the simulations such as saturation magnetization M s =800 kA m −1 , exchange stiffness A ex =13 pJ m −1 , damping constant α =0.01, zero magnetocrystalline anisotropy and a cell size of 3 × 3 × 10 nm 3 . The actual ‘array environment’ for the disks was set up by introducing a periodic boundary condition, where the ‘primary’ sample, a single disk is repeated infinitely many times in the xy plane and all repeated disks have the same magnetization configuration during the dynamic process. We also performed the simulations with different boundary conditions, that is, four disks are used as the ‘primary’ sample and clarified that the boundary condition does not affect the result for the dynamic process of vortex creation depending on the interdisk distance. 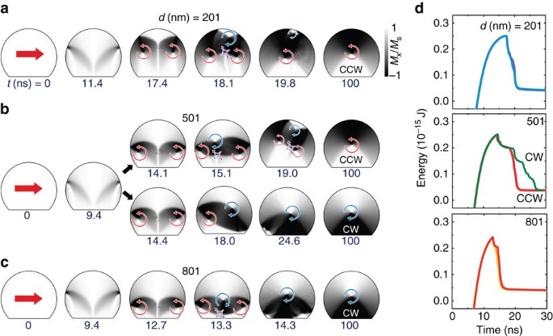Figure 3: Micromagnetic simulations on the dynamic process of VS formation. Simulated images for the dynamic process of vortex formation in the disks within the arrays ofd=201 nm (a),d=501 nm (b) andd=801 nm (c) together with the energy variation during the dynamic process (d). The CCW (CW) circularity is indicated by the red (blue) arrow. The yellow arrow with diamond shape represents the antivortex. In the disks ofd=501 nm, various dynamics patterns are observed in repeated simulations, which were performed under identical conditions. Figure 3 shows simulated images for the formation of VSs in the disks (Fig. 3a–c) together with the variation of total energy during the process (Fig. 3d) taken from the simulation using a periodic boundary condition with a single disk. We have chosen disk arrays of 2 R =999 nm, h =40 nm, r =0.3 R and an interdisk distance of d =201, 501 and 801 nm as model systems, which are closest to the experimental scenario and which can easily be obtained with a 3-nm cell size in the simulations. Further, to mimic the experimental procedure, the disks were saturated by a magnetic field of 1 kOe in the positive x -direction and then directly relaxed by an exponential decay field with a relaxation time of τ =4.4 ns. The dynamics of VS formation in the disks is quite complex. It proceeds with multiple creation and annihilation processes of topological solitons such as vortices having integer winding number, n =±1 and edge solitons having half integer winding number, n =±1/2 (refs 33 , 39 , 40 ) ( Supplementary Note 1 ). It is important to note that the topological charge (total winding number N ) is conserved over the whole process. Figure 3: Micromagnetic simulations on the dynamic process of VS formation. Simulated images for the dynamic process of vortex formation in the disks within the arrays of d =201 nm ( a ), d =501 nm ( b ) and d =801 nm ( c ) together with the energy variation during the dynamic process ( d ). The CCW (CW) circularity is indicated by the red (blue) arrow. The yellow arrow with diamond shape represents the antivortex. In the disks of d =501 nm, various dynamics patterns are observed in repeated simulations, which were performed under identical conditions. Full size image Chaotic dynamics in the vortex formation Interestingly, we found that in the disk of d =501 nm, various dynamic patterns are observed within the repeated simulations even without external stimulators such as thermal noises, whereas the dynamics in the disks of d =201 nm and d =801 nm appears to be completely deterministic. The series of images in Fig. 3b are two representative examples out of a wide variety of dynamic patterns simulated in the case of d= 501 nm ( Supplementary Note 2 ). Although the dynamic processes of VS formation are nearly identical at an early stage, that is, at short timescales (< t =14 ns), they become widely different at a later stage. The sudden fluctuation of dynamics becomes also evident in the total energy variation during the process ( Fig. 3d ). At initial spin configurations, the energy difference in two dynamic cases is very small, Δ E =4.3 × 10 −29 J, but a slight variation of energy at initial state results in the diverging of energy at later time (> t =14 ns). This is a typical characteristic of chaos, where the final outcome is very sensitive to the initial conditions, an effect, which is referred to the ‘butterfly’ effect [41] . The behaviour of classical chaos in the dynamic process of vortex creation has so far not been addressed. Surprisingly, this chaotic dynamics is a particular phenomenon for the disk with d= 501 nm and it is in sharp contrast to the deterministic dynamics seen in the disks with d= 201 nm and d= 801 nm where almost no energy fluctuation exists over the whole process, although the energy difference between two dynamic cases in initial conditions of those disks were on equal levels (~10 −29 J) as for the disk with d =501 nm. It should be noted that each dynamics in Fig. 3b ends up with a different circularity. Consequently, the chaotic dynamics adds stochasticity to the circularity formation by causing the random creation of CW and CCW circularity in a single disk. This is unlike the creation of only one type of circularity in the disk of d= 201 nm or d= 801 nm, either CCW or CW, which corresponds to the majority of each array in the experimental results ( Fig. 2 ). These simulation results strongly support that the chaotic dynamics plays a crucial role for the higher stochasticity in the disks with d =501 nm as observed in the experimental results ( Fig. 2 ). They also suggest that the dynamics itself can be a critical factor for the stochastic nature in the VS formation of asymmetric disks. Further, our simulations prove that the stochasticity occurring in the disks with d =201 and 801 nm is not a consequence of the dynamics as the dynamics in the disks is completely deterministic and the final circularity is identical in all simulations. We conclude that the experimentally observed results of some degree of stochasticity in the disks of d =201 and 801 nm and even in the disks of d =501 nm is a result of thermal fluctuations. Under the influence of extrinsic factors such as roughness and defects, the degree of stochasticity caused by the thermal fluctuation effect could differ from disk (array) to disk (array). However, the experimentally observed V-shaped dependency of stochasticity on the interdisk distance can be only explained by including dynamic aspects, specifically chaotic dynamics. Simulated stray field distributions To explain why the unconventional chaotic dynamics appears only in the disks with a particular interdisk distance, d =501 nm, we took into account the stray fields induced by adjacent disks considering that the magnetic quantity, which most sensitively depend on the interdisk distance in disk arrays, is the strength of stray fields [42] , [43] . 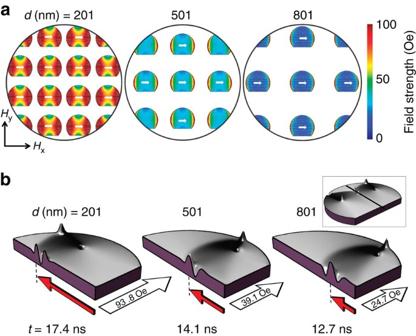Figure 4: Simulated stray field distributions. (a) The distribution of the stray fields induced by adjacent Py disks with saturated magnetization configuration along +xdirection. The white arrow indicates the direction of the stray fields. The strength of stray fields is represented on the colour bar. (b) The magnetization configurations in one half of the disks withd=201, 501 and 801 nm att=17.4, 14.1 and 12.7 ns during the dynamic process. The height on the cross-section and grey scale indicates themzandmxdistributions, respectively. The red arrow indicates how far the vortices are displaced from flat edges of disks at the stage of dynamics. The direction of the stray fields and the strength of stray fields are denoted by white arrows in each disk. Figure 4a represents the distributions of stray fields over the disks of d =201, 501 and 801 nm. All disks have the same saturated magnetization configuration for an external field of 1 kOe pointing in + x direction. As the horizontally generated stray fields are larger than the vertical stray fields, the resultant stray fields point in the direction of + x and are concentrated at the left and right edges of asymmetric disks. We confirmed that for the interdisk distance of d =201, 501 and 801 nm, the average strength of stray fields in the disks drastically decreases such as H de =93.8, 39.1 and 24.7 Oe, respectively, as indicated by the colour code in Fig. 4a . The stray fields are mainly composed of the H x component, whereas the H y component can be ignored. Figure 4: Simulated stray field distributions. ( a ) The distribution of the stray fields induced by adjacent Py disks with saturated magnetization configuration along + x direction. The white arrow indicates the direction of the stray fields. The strength of stray fields is represented on the colour bar. ( b ) The magnetization configurations in one half of the disks with d =201, 501 and 801 nm at t =17.4, 14.1 and 12.7 ns during the dynamic process. The height on the cross-section and grey scale indicates the m z and m x distributions, respectively. The red arrow indicates how far the vortices are displaced from flat edges of disks at the stage of dynamics. The direction of the stray fields and the strength of stray fields are denoted by white arrows in each disk. Full size image Looking into the details of the dynamic process in each array, which has different strengths of stray fields, we found that the location of vortices during the dynamic process is very crucial in the determination whether the dynamics will be chaotic or deterministic. In Fig. 4b , we show the magnetization configurations in one half of disks with d =201, 501 and 801 nm at t =17.4, 14.1 and 12.7 ns during the dynamic process shown in Fig. 3 . The cross-section plane is taken from the vertical centreline as indicated in the inset. The height along the cross-section and grey scale indicates the m z and m x profiles over the half of disks, respectively. As shown by red arrows representing how far the vortices are vertically displaced from the flat edges of disks at the time, the position of vortices sensitively depends on the strength of the acting stray fields. The vortices are near the top and bottom edges of disks at the stray fields of 93.8 and 24.7 Oe in the disks of d =201 and 801 nm, respectively. However, they are located in the centre of the disk vertically at the stray fields of 39.1 Oe in the disks of d =501 nm. As a result of the vortices’ positions near the top or bottom edge of the disk, the dynamic process continues to proceed in a deterministic way as seen in Fig. 3a,c . Namely, in the disks of d =201 ( d =801 nm) with strong (weak) stray fields, the CW (one CCW) vortex near the top (flat) edge of disk disappears with the two edge solutions and one CCW (the second CCW) vortex annihilates with the antivortex ( Supplementary Note 1 ). Finally, the second CCW (the CW) vortex located in inner disk remains in the disks of d =201 nm (801 nm). The remaining CCW (CW) vortex becomes the eventual VS with well-defined circularity in the disk of d =201 nm (801 nm). On the other hand, the location of vortices at intermediate strength of the stray fields, 39.1 Oe, in the disk of d =501 nm leads to the chaotic dynamics. As dynamics proceeds, vortices located in the vertical centre of disk can move either up or down yielding the dynamic pattern for CCW or CW circularity. Tuning the stray field strength with the interdisk distance in asymmetric disks one can therefore completely control the stochastic nature dictated by the chaotic dynamics. In conclusion, the origin of our experimental observation of stochastic nucleation of circularity in magnetic vortices is explained by micromagnetic simulations, which provide evidence that the chaotic dynamics in the initial stages of vortex formation on an ultrafast timescale can trigger the stochastic behaviour at steady state in asymmetric disk arrays. Our work not only demonstrates that dynamic itself can be a decisive factor causing the stochastic behaviour but also it shows the possibility to control the ‘intrinsic’ stochastic nature in the vortex creation process. Sample preparation and MTXM measurement Polycrystalline permalloy (Py) disks with a flat edge were patterned by electron-beam lithography and lift-off processing. The radius and thickness of disks were fixed as 2 R =1 μm and t =40 nm, respectively, and the edge rate was varied from r =0.1 R to 0.3 R . The arrays consisting of 30 × 30 asymmetrically shaped disks with different interdisk distances of d =200, 500 and 800 nm were deposited on 100-nm-thick silicon-nitride membranes, which allow sufficient X-ray transmission. The VSs in Py disks were directly observed utilizing full-field MTXM at the Advanced Light Source (XM-1, beamline 6.1.2) [34] . Individual images consisting of tens of disks can thus be taken within seconds. The large field of view (~8 μm) at XM-1 allowed accumulating high statistical accuracy by repeated measurements of 25 disks out of total 900 disks. The optical setup for XM-1 is described elsewhere [44] . It consists of two Fresnel zone plates used as condenser and objective lens, which allows to record real space images with high lateral resolution down to currently 25 nm. Using circularly polarized X-rays, beam magnetic contrast is provided by X-ray magnetic circular dichroism. As the X-ray magnetic circular dichroism signal is proportional to the projection of the magnetization vector along the photon momentum direction, in-plane spin configurations can be recorded by mounting the samples at 60° with respect to the X-ray propagation direction. The magnetic imaging in Py disks was carried out at the Fe L 3 X-ray absorption edge at 707 eV. External magnetic fields up to 2 kOe can be applied during the image acquisition. How to cite this article: Im, M.-Y. et al. Stochastic formation of magnetic vortex structures in asymmetric disks triggered by chaotic dynamics. Nat. Commun. 5:5620 doi: 10.1038/ncomms6620 (2014).